Disk-cylinder and disk-sphere nanoparticles via a block copolymer blend solution construction Researchers strive to produce nanoparticles with complexity in composition and structure. Although traditional spherical, cylindrical and membranous, or planar, nanostructures are ubiquitous, scientists seek more complicated geometries for potential functionality. Here we report the simple solution construction of multigeometry nanoparticles, disk-sphere and disk-cylinder, through a straightforward, molecular-level, blending strategy with binary mixtures of block copolymers. The multigeometry nanoparticles contain disk geometry in the core with either spherical patches along the disk periphery in the case of disk-sphere particles or cylindrical edges and handles in the case of the disk-cylinder particles. The portions of different geometry in the same nanoparticles contain different core block chemistry, thus also defining multicompartments in the nanoparticles. Although the block copolymers chosen for the blends are important for the definition of the final hybrid particles, the control of the kinetic pathway of assembly is critical for successful multigeometry particle construction. Compositional and geometrical complexity of nano-sized objects has long been an important topic in materials science leading to novel properties and applications in fields such as nano-medicine [1] , organic photonics [2] and electronics [3] . Beyond the considerable success in confining multiple materials and compositions into nano-objects with simple geometric shapes such as spheres, cylinders and vesicles [4] , [5] , [6] , [7] , recent attention has focused on the impact of particle geometry on optical [8] , electronic [9] and biomedical [10] properties. However, a systematic understanding of nanoparticle construction with both compositional and geometrical complexity does not yet exist. Nano-objects have been successfully constructed via solution supramolecular assembly from a wide range of multi-component molecular building units, such as block copolymers [5] , [6] , [7] , block copolypeptides [11] and DNA [8] , with well-defined structures and functions manipulated by constituent molecular architecture and component chemistry. Block copolymers consist of two or more chemically different polymer components linked together by covalent bonding. Block copolymer molecules form specific geometries of solution-assembled, micelle-like nanoparticles determined by the relative volume of the respective blocks, the interaction between polymer block segments and the interaction of the respective blocks with the solvent ( Fig. 1a,b ) [12] . In a solvent that selectively solubilizes one block of a block copolymer, molecules aggregate predominately into bilayer membranes (that is, vesicles), cylinders or spheres. Nanostructure geometry can be controlled precisely by changing the relative block lengths, by adding external stimuli such as solvent mixing [5] or addition of other molecules that specifically associate with and tune a desired block volume in an assembly [13] , [14] , and by changing the solvent processing kinetic pathway [15] , [16] . Owing to the slow molecular exchange dynamics between block copolymer assemblies and the solvent that prevents global thermodynamic equilibration [17] , nanoparticles with kinetically trapped, complex nanostructures are achievable. 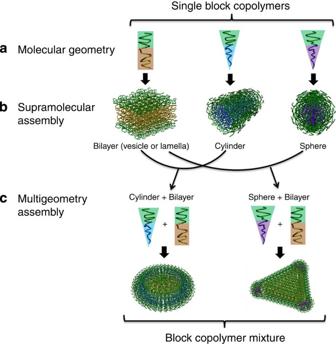Figure 1: Schematic design for multigeometry nanoparticle construction. Single block copolymers possess (a) specific molecular geometries based on relative length of block and solvophilicity/solvophobicity of the respective blocks. The individual block copolymers can assemble into (b) bilayer membranes (for example, vesicles), cylinders or spheres, through desired solution assembly. By taking advantage of molecular design and synthesis, varied block copolymers are assembled into diverse geometries at the same assembly condition. Herein, (c) multigeometry nanoparticles are achievable from co-assembly of selected mixtures of block copolymers in unlike molecular geometries, for example, cylinder-forming and bilayer-forming block copolymer mixture, or sphere-forming and bilayer-forming block copolymer mixture. Figure 1: Schematic design for multigeometry nanoparticle construction. Single block copolymers possess ( a ) specific molecular geometries based on relative length of block and solvophilicity/solvophobicity of the respective blocks. The individual block copolymers can assemble into ( b ) bilayer membranes (for example, vesicles), cylinders or spheres, through desired solution assembly. By taking advantage of molecular design and synthesis, varied block copolymers are assembled into diverse geometries at the same assembly condition. Herein, ( c ) multigeometry nanoparticles are achievable from co-assembly of selected mixtures of block copolymers in unlike molecular geometries, for example, cylinder-forming and bilayer-forming block copolymer mixture, or sphere-forming and bilayer-forming block copolymer mixture. Full size image The ability to kinetically trap block copolymers into nanoparticles and observe local equilibration within the particles provides an excellent opportunity to construct complex, multi-component nano-objects for multifunctional, hierarchical materials [18] , [19] . In single diblock copolymer solution suspensions, assemblies with locally mixed geometries, for example, cylinders with sphere end-caps and Y-junctions between cylinders, have been found at relative block compositions that lie between molecular compositions that form traditional spheres and cylinders or cylinders and vesicles [20] . In blends of different block copolymers with identical block chemistry but different block lengths, cylinders with sphere end-caps and vesicles with cylinder branches have been observed due to the local trapping and segregation of block copolymers with different molecular weights [21] . Alternately, one can purposely mix different block copolymers with unlike block chemistries into multi-component nanoparticles with proper kinetic processing. The limited examples of this strategy have focused on block copolymer molecules with similar molecular weights and relative block fractions for the production of blended spheres [22] , [23] , cylinders that contain multiple block copolymers [15] , [23] , [24] , [25] and blended vesicles [26] , [27] . Here, we develop a straightforward solution processing strategy for multigeometry nanoparticle construction that produces hybrid geometry, disk-sphere or disk-cylinder polymeric nanoparticles. Final multi-geometry nanoparticles are part disk and either part cylinder or part sphere and are formed simply through blending of two unlike block copolymers into mixed nanoparticles that subsequently segregate locally into sub-domains of distinct geometry and distinct core block chemistry. We show that this strategy can be used to construct novel soft matter nanostructures with designed compositions and geometries from simple block copolymers. Multigeometry discoid assembly strategy In this present work, nanoparticles with hybrid discoid morphologies have been constructed with mixed block copolymers assembled through kinetic control in solution. Rather than closing into vesicles, disks [28] , [29] are flat bilayer sheets that are restricted to finite size. Due to inherent geometrical anisotropy, discoid structures exhibit notable shear field-responsive capabilities for prolonged discoid particle blood circulation time [30] , are used for membrane protein structure determination via 1 H NMR spectroscopy [31] , are used as templates for drug delivery [32] and for porous material construction [33] . The difficulty in bilayer disk assembly is that the rim around the edge of a discrete disk is a high energy defect; to avoid the exposure of hydrophobic block to the aqueous medium, the molecules around the edge may rearrange to adopt a much higher curvature, as opposed to the flat interfacial curvature that the molecules favour throughout the interior of the nanoparticle [34] ( Supplementary Fig. S1 ). An approach to form disk structures is to cut vesicles into disks through blending with other block copolymer molecules that prefer to adopt a higher interfacial curvature after assembly in order to stabilize a disk edge. One successful small molecule example of this blending strategy is the formation of discoid bicelles through the mixing of long-chain phospholipids that form planar bilayers surrounded by short-chain lipids on the edge that shield the long-chain lipid-tails from water [35] . With proper design of block components and lengths, macromolecular block copolymers exhibit diverse morphologies at the same solution condition, that is, vesicle, cylinder or sphere, where molecules express increasing interfacial curvature, respectively ( Fig. 1 ). Therefore, new, multigeometry disk nanoparticles were achievable from solution co-assembly of a bilayer-forming block copolymer and a cylinder-forming or sphere-forming block copolymer, respectively. Disk-cylinder hybrid nanoparticles Both molecules of the designed binary block copolymer blends presented here possessed the same poly(acrylic acid) (PAA) hydrophilic block chemistry with similar block lengths but possessed different, incompatible hydrophobic blocks, that is, polystyrene (PS) or polyisoprene (PI). 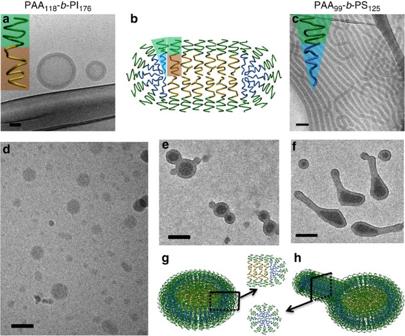Figure 2: Disk-cylinder multigeometry nanoparticles. Block copolymer(s) were assembled in a THF and water solvent mixture (20 v% THF, 80 v% H2O) in the presence of EDDA at an amine-to-acid ratio=0.5. (a) Cryo-TEM image of vesicles formed by PAA118-b-PI176. (b) Cross-sectional schematic shows the desired organization of block copolymer molecules into disk assemblies. (c) Cryo-TEM image of cylindrical micelles formed by PAA99-b-PS125. (d) Cryo-TEM image and (e,f). OsO4stained TEM images of hybrid particles formed by equal molar blend of PAA118-b-PI176and PAA99-b-PS125; (f) shows the formation of the minority component tailed-disk structure. Proposed distributions of block copolymer molecules in the disk and tailed-disk assemblies are illustrated in (g,h). EDDA molecules that closely associate with the PAA blocks within the assembled nanoparticles are not shown in the schematics for clarity. Scale bar, 100 nm. Figure 2 displays the circular, disk-like nanoparticles assembled through a defined tetrahydrofuran (THF) and water solvent-mixing pathway ( vide infra ) from an equal molar blend of PAA 118 - b -PI 176 (the subscripts refer to the number-averaged degrees of polymerization) and PAA 99 - b -PS 125 diblock copolymers in the presence of small, di-functional organoamines, 2,2′-(ethylenedioxy)diethylamine (EDDA). Mixed with the same amount of EDDA diamines at an amine-to-acid ratio of 0.5, neat PAA 118 - b -PI 176 and neat PAA 99 - b -PS 125 assembled into vesicles ( Fig. 2a ) and cylindrical micelles ( Fig. 2c ), respectively, at high water content (20 v% THF, 80 v% H 2 O). The thickness of the vesicular membrane and cylinder diameter as measured from an average of 100 particles in cryo-TEM were 35±3 nm and 33±2 nm, respectively. Upon co-assembly of the two diblock copolymers with EDDA at the same amine-to-acid ratio of 0.5, circular particles with diameter ≤100 nm were formed with homogeneous contrast in cryo-TEM imaging, Fig. 2d , indicative of the formation of flat, disk-like nanostructures. The co-existing oblate and needle-like structures result from disk particles at different orientations with respect to the electron beam. The morphology was further confirmed by OsO 4 staining in cast films of the nanoparticles collected from the same sample solution ( Fig. 2e , OsO 4 selectively stained PI by reacting with carbon double bonds). A dark, central, flat region is where the PAA- b -PI molecules were observed in each particle, surrounded by a grey rim area rich in PAA- b -PS. A minor population of larger particles (size >100 nm, Fig. 2f ) was observed with a grey cylindrical PAA- b -PS tail extending out of the disk. The width of the disk rim was constant, approximately half of the diameter of the PAA- b -PS cylinder tails, suggesting a half cylinder of PAA- b -PS molecules packing around PAA- b -PI bilayer as illustrated in Fig. 2g,h . Additional cryo-TEM and cast-film data of disk-cylinder hybrid particles are shown in Supplementary Figs S3,S4 , respectively. Figure 2: Disk-cylinder multigeometry nanoparticles. Block copolymer(s) were assembled in a THF and water solvent mixture (20 v% THF, 80 v% H 2 O) in the presence of EDDA at an amine-to-acid ratio=0.5. ( a ) Cryo-TEM image of vesicles formed by PAA 118 -b-PI 176 . ( b ) Cross-sectional schematic shows the desired organization of block copolymer molecules into disk assemblies. ( c ) Cryo-TEM image of cylindrical micelles formed by PAA 99 - b -PS 125 . ( d ) Cryo-TEM image and ( e , f ). OsO 4 stained TEM images of hybrid particles formed by equal molar blend of PAA 118 -b-PI 176 and PAA 99 - b -PS 125 ; ( f ) shows the formation of the minority component tailed-disk structure. Proposed distributions of block copolymer molecules in the disk and tailed-disk assemblies are illustrated in ( g , h ). EDDA molecules that closely associate with the PAA blocks within the assembled nanoparticles are not shown in the schematics for clarity. Scale bar, 100 nm. Full size image The morphology of each disk-cylinder hybrid particle was defined by the materials trapped inside. As shown in Fig. 3 , small particles in diameter of ~50 to 80 nm possessed a round discoid membrane of PAA- b -PB and a half cylinder rim of PAA- b -PS. As particle size increased, the PAA- b -PB membrane generally elongated into oblate disk for an increased rim area to pack more PAA- b -PS half cylinders around the edge. With even more PAA- b -PS trapped in a particle, full cylinders would form and extend out from the oblate disks. By simply comparing the relative areas of dark (PI-containing block copolymer) to light (PS-containing block copolymer) in the hybrid particle population, the volume ratio of PS to PI in the particles overall well represent the equimolar ratio of the two block copolymers in the initial blend of PAA- b -PS and PAA- b -PI. 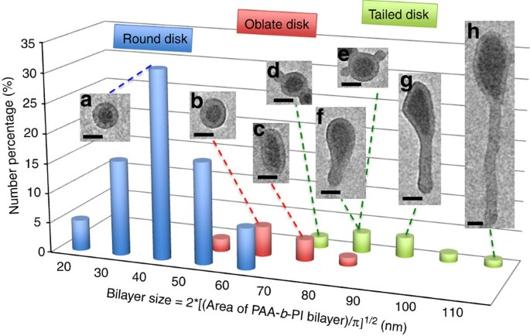Figure 3: Statistical evaluation of disk-cylinder hybrid morphologies. Column graph shows the number percentage of disk-cylinder multigeometry nanoparticles of slightly different morphology (produced from analysis of 100 particles in OsO4stained TEM image). Blue, red and green columns are corresponding to populations of round disk, oblate disk and tailed-disk, respectively. The sizes of the bilayer section of the particles were calculated from the area of dark PAA-b-PI disk region in the particles by an equation of bilayer size=2*[(Area of PAA-b-PI bilayer)/π]1/2. The bilayer size is equal to the diameter of the central dark region of PAA-b-PI assuming a round disk section to simply give a measure of size comparison between particle disk sections. Insert images are OsO4stained TEM showed the selected particle morphologies in the same sample of round disk (a), oblate disks (b,c) and tailed disks (d–h) of different bilayer sizes indicated by dash lines. Scale bar, 50 nm. Figure 3: Statistical evaluation of disk-cylinder hybrid morphologies. Column graph shows the number percentage of disk-cylinder multigeometry nanoparticles of slightly different morphology (produced from analysis of 100 particles in OsO 4 stained TEM image). Blue, red and green columns are corresponding to populations of round disk, oblate disk and tailed-disk, respectively. The sizes of the bilayer section of the particles were calculated from the area of dark PAA-b-PI disk region in the particles by an equation of bilayer size=2*[(Area of PAA- b -PI bilayer)/π] 1/2 . The bilayer size is equal to the diameter of the central dark region of PAA-b-PI assuming a round disk section to simply give a measure of size comparison between particle disk sections. Insert images are OsO 4 stained TEM showed the selected particle morphologies in the same sample of round disk ( a ), oblate disks ( b , c ) and tailed disks ( d – h ) of different bilayer sizes indicated by dash lines. Scale bar, 50 nm. Full size image The success in multigeometry assembly from block copolymer mixtures relies on two phenomena: proper nanoparticle confinement and subsequent internal organization. Kinetic control of the assembly process through the proper solvent-mixing pathway is critical for success with proper nanoparticle confinement. The solvent-mixing pathway began with dissolution of a desired amount of block copolymers mixed with EDDA diamines in THF. THF is a good solvent for the block copolymers, while the EDDA complexes with the PAA blocks to form cores of inverse micelle-like aggregate structures. Subsequent addition of water had the combined effect of aggregating the hydrophobic blocks into new nanoparticle hydrophobic cores, while concurrently swelling PAA-EDDA complexed hydrophilic blocks into the new nanoparticle shells. Final micelle-like nanoparticles were obtained when water addition reached a volume ratio of 4:1 water to THF. The complexation of the EDDA amines with PAA acid groups impacted the final morphology in two critical aspects. First, the amines help to tune the shell volumes of the final assembly and thus define the geometry of nanoparticle that a block copolymer would like to adopt [26] . Second, the initial complexation of the PAA and amines in pure THF forces the different block copolymers to reside in the same nanoparticles during assembly, consequently producing particles with mixed hydrophobic cores at higher water content that undergo local, internal phase separation to form multigeometry particles. Obviously, the assembly conditions (solvent composition, block molecular weight, amount and type of amine) must provide for dynamic behaviour within the formed nanoparticles so that local phase separation of unlike hydrophobic blocks can produce the final, multigeometry nanoparticles. Block copolymer blends in an absence of diamines assembled into two separate, ill-defined nanoparticle phases of the two respective diblock copolymers due to the lack of initial confinement in the same nanoparticle in neat THF ( Supplementary Fig. S2 ). In addition, assembly with excessive addition of diamines (amine-to-acid ratio >1.0) produced only spherical nanoparticles for both block copolymers at the desired solution mixture. Therefore, we narrowed the studied amine-to-acid ratio to between 0.3 and 1.0 in order to find appropriate conditions for desired, different particle geometries to be blended into the same nanoparticle with kinetic control. An additional critical aspect of the multigeometry particle assembly strategy is that the presence of the amine-acid complexation and the large molecular weight of the block copolymers both serve to significantly slow chain exchange with the solvent [17] . All of these effects, together, explain why block copolymer chains phase segregate and equilibrate locally within the same nanoparticle. This intraparticle segregation results in the highly interesting and unique expression of the respective block copolymer preferred bilayered or cylindrical geometries within the same nanoparticle. Disk-sphere hybrid nanoparticles Through this kinetically controlled assembly strategy, sphere-forming block copolymer was also forced to assemble with a vesicle-forming block copolymer and form disk-sphere hybrid nanoparticles. Under the same solution assembly conditions as the vesicle-cylinder blend vide supra , a vesicle-forming triblock copolymer PAA 150 - block -poly(methyl acrylate) 60 - block -PS 240 (PAA 150 - b -PMA 60 - b -PS 240 ) and a sphere-forming diblock PAA 75 - block -polybutadiene 104 (PAA 75 - b -PB 104 ) were blended at a 4:1 molar ratio to produce disk-sphere multigeometry nanoparticles as shown in Fig. 4 and Supplementary Fig. S5 . The triblock and diblock copolymers possessed the same PAA block chemistry but different hydrophobic blocks. A large difference from the earlier disk-cylinder blend is that the lengths of the respective hydrophilic or hydrophobic blocks of the two block copolymers were substantially different. The thickness of the vesicular membranes and sphere diameter as measured from an average of 100 particles in cryo-TEM were 54±5 nm and 32±5 nm, respectively, in the samples of the individual block copolymers ( Fig. 4a,c ). In the OsO 4 stained cryo-TEM images ( Fig. 4d , OsO 4 selectively stained PB by reacting with double bonds), disk nanoparticles with a broad range of sizes (50–300 nm) and number of hemispherical caps (1–6, Fig. 4e–j ) were obtained simultaneously. The hybrid particle formation was achieved owing to combined contributions from both PAA- b -PB and PAA- b -PMA- b -PS to stabilize the rim area: sphere-forming PAA- b -PB aggregated into hemi-spheres capping the edge apices of the disks, whereas the remaining edge boundaries between the hemispherical caps consisting of PAA- b -PMA- b -PS tended to be straight, thus limiting the length of higher energy disk edge defect. The original blend ratio is qualitatively observed in the more dominant population of small particles. In larger particles, there is much more disk formation in the hybrid disk-sphere particles. There appears to be a maximum number of sphere caps per disk edge distance that is stable in the larger hybrid particles. Therefore, the excess PAA- b -PB must be aggregated into spherical particles that have broken away from the hybrid particles (see the many, very small particles in Fig. 4d ). The PAA- b -PMA- b -PS molecules at the disk straight edges between the hemispherical caps adopt frustrated packing at the edge, as illustrated in Fig. 4b . This frustrated packing shields the hydrophobic core of the disk from solvent, as the hybrid particles do not aggregate together, as would be expected if there were exposed hydrophobic edges. 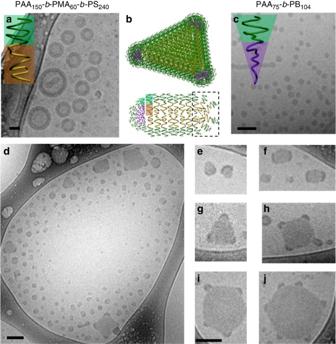Figure 4: Disk-sphere multigeometry nanoparticles. Block copolymer(s) were assembled in a THF and water solvent mixture (20 v% THF, 80 v% H2O) in the presence of EDDA at an amine-to-acid ratio=0.5. (a) Cryo-TEM image of vesicles formed by PAA150-b-PMA60-b-PS240. (c). Cryo-TEM image of spherical micelles formed by PAA75-b-PB104. (d) OsO4stained cryo-TEM image of hybrid particles formed by 4:1 molar ratio blend of PAA150-b-PMA60-b-PS240and PAA75-b-PB104. (e–j) OsO4stained cryo-TEM images show the selected disk-sphere multigeometry nanoparticles with 1–6 sphere caps on the disk edges. Proposed distributions of block copolymer molecules in the hybrid nanoparticles are illustrated in (b). PAA150-b-PMA60-b-PS240also reside in the disk rim area between spherical edge caps of PAA75-b-PB104as marked by the dashed square. PMA and PS hydrophobic blocks are both coloured gold for clarity. EDDA molecules that closely associate with the PAA blocks within the assembled nanoparticles are not shown in the schematics for clarity. Scale bar, 100 nm. Figure 4: Disk-sphere multigeometry nanoparticles. Block copolymer(s) were assembled in a THF and water solvent mixture (20 v% THF, 80 v% H 2 O) in the presence of EDDA at an amine-to-acid ratio=0.5. ( a ) Cryo-TEM image of vesicles formed by PAA 150 - b -PMA 60 - b -PS 240 . ( c ). Cryo-TEM image of spherical micelles formed by PAA 75 - b -PB 104 . ( d ) OsO 4 stained cryo-TEM image of hybrid particles formed by 4:1 molar ratio blend of PAA 150 - b -PMA 60 - b -PS 240 and PAA 75 - b -PB 104 . ( e – j ) OsO 4 stained cryo-TEM images show the selected disk-sphere multigeometry nanoparticles with 1–6 sphere caps on the disk edges. Proposed distributions of block copolymer molecules in the hybrid nanoparticles are illustrated in ( b ). PAA 150 - b -PMA 60 - b -PS 240 also reside in the disk rim area between spherical edge caps of PAA 75 - b -PB 104 as marked by the dashed square. PMA and PS hydrophobic blocks are both coloured gold for clarity. EDDA molecules that closely associate with the PAA blocks within the assembled nanoparticles are not shown in the schematics for clarity. Scale bar, 100 nm. Full size image In summary, we used a molecular-level geometric blending strategy for complex block copolymer nanoparticle construction with designed compartments and multiple geometries. Disk-cylinder and disk-sphere multigeometry nanoparticles have been obtained through the simple solvent-mixing process. With further exploration in size and shape, variety of the molecular units and further advancement in kinetic control and solution processing, more well-defined, complex multigeometry nanoparticles are expected from new, binary, ternary or higher order blends with desired relative amount of each component and potential multifunction. In addition to the attractive shapes and complex morphologies that these multigeometry nanostructures possess globally, the local differentiation of composition leads to segregation of physical, chemical and mechanical properties within a single nanoscopic framework. Advanced investigation of the sub-nanoparticle properties and the incorporation of functional sub-units is expected to lead to highly sophisticated materials that may serve as components for future technological device construction. Sample preparation Block copolymers mixed at certain blending ratio first were dissolved in THF to produce a 0.1 weight per cent homogeneous solution of block copolymer. Next, EDDA was added to give a desired amine-to-acid molar ratio (for example, 0.5:1.0) and to form inverse-like micelle aggregates. Subsequent water addition was performed by slow water titration performed on a syringe pump stage (KD Scientific Syringe Pump, KDS 100). One millilitre Water per hour was added to 0.5 ml THF polymer solution with vigorous stirring. Afterwards, sample solutions were sealed in vials and aged for 1 day before characterization. Transmission electron microscopy TEM imaging was performed on a Tecnai G2 12 microscope operating at an accelerating voltage of 120 kV. TEM samples were prepared by applying a drop of polymer solution (about 2–4 μl) onto a carbon-coated copper TEM grid and allowing the solvents to evaporate under ambient conditions. Images were collected on a Gatan CCD. Cryogenic transmission electron microscopy A Gatan cryo-holder system was used to examine the samples in a Tecnai G2 12 microscope at voltage 120 kV. Sample preparation was performed in the Vitrobot virtrification system. A droplet of the sample solution (10 μl) was dipped on a lacey carbon-coated copper TEM grid. The specimen was blotted and plunged into a liquid ethane container cooled by liquid nitrogen. The vitrified samples were transferred to a Gatan 626 cryo-holder and cryo-transfer stage cooled by liquid nitrogen. During TEM observation, the cryo-holder was maintained below −170 K to prevent the sublimation of vitreous water and THF. The digital images were collected by Gatan low-dose CCD. Staining methods A vapour staining method was applied to cast-film TEM samples. Dried TEM grids were placed on a 25 × 75 × 1 mm 3 glass slide to sit in a sealed 100 ml glass bottle suspended above 1 ml 4 wt% osmium tetroxide aqueous solution (purchased from Electron Microscopy Sciences). OsO 4 vapour staining process lasted from 6–24 h for different samples. A solution staining method was applied to cryo-TEM samples by directly mixing 20 μl 4 wt% osmium tetroxide aqueous solution with 1 ml assembly sample solution upon gird preparation and imaging. Synthesis of PAA- b -PS diblock copolymer The PAA- b -PS diblock copolymer used in this study were synthesized by atom transfer radical polymerization, following previous reported procedures [36] . Briefly, t- butyl acrylate ( ca . 200 equiv.) was polymerized by using ethyl 2-bromopropionate ( ca . 1.0 equiv.) as initiator, CuBr ( ca. 1.9 equiv.) and CuBr 2 ( ca. 0.1 equiv.) as catalysts and N , N , N′ , N′ , N′′ - pentamethyldiethylenetriamine (PMDETA, ca. 2.0 equiv.) as ligand. Polymerization was performed at 50 °C and monitored by withdrawing small aliquots for GPC and 1 H NMR analyses. P t BA 99 was then extended into P t BA 99 - b -PS 125 by chain extension polymerizing with styrene ( ca . 500 equiv. ), using CuBr ( ca . 3.0 equiv.) and PMDETA ( ca . 3.0 equiv.) as catalyst and ligand, at a temperature of 55 °C. The polymerization reactions were quenched at styrene conversion of 25% by freezing in liquid nitrogen. The t- butyl-protected diblock copolymer were then transformed into PAA 99 - b -PS 125 by reacted with iodotrimethylsilane ( ca. 3.0 equiv.) following a reported deprotection protocol [14] . The molecular characteristics of the diblock copolymer is listed in Table 1 . Table 1 Molecular Characteristics of diblock copolymer used in this study. Full size table Synthesis of PAA- b -PI diblock copolymers The precursor PI- b -P t BuA for producing well-defined PAA- b -PI diblock copolymers used in this study were synthesized by anionic polymerization of isoprene and tert- butyl acrylate employing high vacuum techniques according to standard protocol [37] , [38] . Tert -Butyl groups of P t BA blocks were cleaved by mild hydrolysis as reported previously [37] . PI: M n =1.2 × 10 4 g mol −1 (SEC-LLS), PDI, 1.05; PI- b -P t BA: M n =2.3 × 10 4 g mol −1 (SEC), PDI, 1.19. Molar ratio isoprene/acrylic acid=1.5:1 by 1 H NMR. Synthesis of PAA- b -PMA- b -PS triblock copolymers The PAA 150 - b -PMA 60 - b -PS 240 used in this study was synthesized by an atom transfer radical polymerization, following previous reported procedure [39] . In brief, t- butyl acrylate ( ca . 400 equiv.) was polymerized by using ethyl 2-bromopropionate ( ca . 1.0 equiv.) as initiator, CuBr ( ca. 1.9 equiv.) and CuBr 2 ( ca. 0.1 equiv.) as catalysts, and PMDETA ( ca. 2.0 equiv.) as ligand. Polymerization was performed at 50 °C and monitored by withdrawing small aliquots for GPC and 1 H NMR analyses. P t BA 150 was then extended into P t BA 150 - b -PMA 60 by chain extension polymerizing with methyl acrylate ( ca . 500 equiv. ), using CuBr ( ca . 3.0 equiv.) and PMDETA ( ca . 3.0 equiv.) as catalyst and ligand, at a temperature of 55 °C. P t BA 150 - b -PMA 60 was used as a macroinitiator, to extend into P t BA 150 - b -PMA 60 - b -PS 240 , by using CuBr (ca. 3.0 equiv.) as catalysts, and bipyridine (ca. 4.0 equiv.) as ligand, at the temperature of 60 °C. P t BA 150 - b -PMA 60 - b -PS 240 was transformed into PAA 150 - b -PMA 60 - b -PS 240 by reaction with iodotrimethylsilane (ca. 3.0 equiv.). The molecular characteristics of the triblock copolymer is listed in Table 2 . Table 2 Molecular Characteristics of triblock copolymer used in this study. Full size table PAA- b -PB diblock copolymers PAA- b -PB diblock copolymer was purchased from Polymer Source, Inc. and used as received. Composition and molecular weight were tested by 1 H NMR: PAA(5450)- b -PB(5600), PDI=1.10 as indicated by the company. Others EDDA was purchased from Sigma-Aldrich Corporation. THF was purchased from Acros Organics. How to cite this article: Zhu, J. et al . Disk-cylinder and disk-sphere nanoparticles via a block copolymer blend solution construction. Nat. Commun. 4:2297 doi: 10.1038/ncomms3297 (2013).